Biologically inspired achromatic waveplates for visible light Waveplates are planar devices used in optics and optoelectronics to change the polarization state of light. Made of anisotropic dielectric materials such as crystals and thin films, waveplates are not known to exhibit achromatic performance over the visible regime. Inspired by the microvillar structure of R8 cells functioning as polarization converters in the eyes of stomatopod crustaceans, we conceived, designed, fabricated and tested periodically multilayered structures comprising two different types of arrays of nanorods. Morphologically analogous to the ocular cells, here we show that the periodically multilayered structures can function as achromatic waveplates over the visible regime. The tip of the electric field vector of a light wave vibrates in a plane, describing a figure that can vary in shape from a straight line to a circle to an ellipse. Accordingly, light is said to be either linearly polarized or circularly polarized or, in general, elliptically polarized. Elliptically polarized light has two linearly polarized components, the electric field vectors of which are mutually orthogonal and can have a phase difference. For any polarization state, another polarization state can be found such that the two are mutually orthogonal. The conversion of one polarization state into another is a key manipulation in optical science and engineering. A waveplate alters the polarization state of light passing through it by creating a relative phase between the linearly polarized components [1] , [2] , [3] . A typical waveplate is a plate made of an anisotropic dielectric material [4] —either a natural crystal such as calcite and quartz [2] or a thin film [5] , [6] —which displays birefringence, by presenting different refractive indexes to the two linearly polarized components of incident light [7] . The difference in the two refractive indexes, being wavelength dependent in general, leads to wavelength-dependent retardation of the phase of one polarization state in relation to that of the orthogonal polarization state. But a desirable waveplate must transmit light of a fixed polarization state uniformly over a broad range of wavelengths. Achromatic performance requires the waveplate to be made of a material whose intrinsic optical properties compensate other wavelength-dependent effects. Furthermore, the transmittance must be sufficiently high and weakly dependent on the wavelength for a waveplate to be useful. Achromatic waveplates are needed for three-dimensional displays [8] and CD/DVD readers [9] , among several optical applications. But a suitable quartz waveplate, besides being fragile due to ∼ 15-μm thickness, exhibits considerable variation in phase retardation over the entire visible regime (400–700 nm wavelength range) [10] , and elaborate designs are needed even for partial success [10] , [11] , [12] , [13] , [14] . A recent study has demonstrated the presence of achromatic waveplates in the eyes of stomatopod crustaceans of species Odontodactylus scyllaru [15] . Comprising many eyelets or ommatidia, each compound eye of such stomatopod crustaceans can distinguish the left-handed or right-handed circular polarized light that is emitted as a sexual signal from a male or female [15] . The key to this discrimination is the exceptionally sophisticated morphology of the R8 cell of each ommatidium. An array of aligned microvilli in the R8 cell functions as a quarter waveplate, better than engineered waveplates [10] . The effective birefringence displayed by the microvillar array has two components: intrinsic birefringence of the microvilli material and form birefringence from the aciculate (that is, needle-like) geometry of the microvilli. The subwavelength optical architecture of the cellular structure thus integrates two dispersive mechanisms for birefringence to deliver a wavelength-independent phase retardation over the visible regime. Fabrication of this subwavelength nanostructure could yield achromatic waveplates (and other optical devices) for operation throughout the visible regime. A biologically inspired artificial achromatic waveplate designed and fabricated as a periodic multilayer structure (PMS) with a unit cell made of two different nanorod arrays fabricated with two different physical vapour deposition methods [5] , [16] , [17] , [18] is reported here. The first method, called the oblique angle deposition (OAD) method [5] , [16] , requires the production of a collimated vapour that collects on a planar substrate as an array of parallel and tilted nanorods owing to a self-shadowing effect. This array of nanorods is effectively a dielectric thin film, which is biaxially anisotropic, because the nanorods are aciculate and have non-circular cross-section [17] , [18] . The second method is called the serial bideposition (SBD) method, wherein two collimated vapors are produced sequentially and sufficiently rapidly so that the nanorods are upright [18] , [19] , [20] ; hence, the thin film exhibits an enhanced refractive index difference in relation to the one produced with only one collimated vapour [19] , [20] . Tantalum oxide (Ta 2 O 5 ) was chosen for both OAD and SBD methods because its refractive index is almost constant over the visible regime, and also it is chemically and thermally stable [21] , [22] , [23] , [24] . 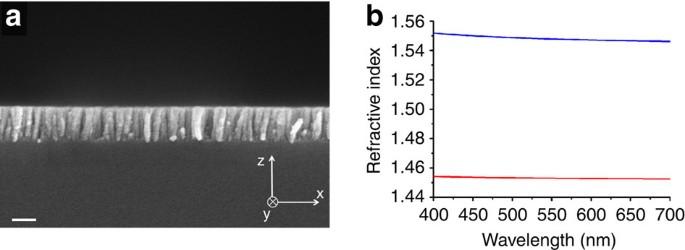Figure 1: The structure and equivalent refractive indexes of a serial bideposited Ta2O5nanorod array. (a) Cross-sectional scanning electron micrograph of an array of upright Ta2O5nanorods produced using the SBD method. Each collimated vapour produced a 5-nm growth, the total thickness of the nanorod array being 174±5 nm. Scale bar, 100 nm. (b) Equivalent refractive indexesnx(red line) andny(blue line) of this array in the visible regime. Birefringence of a serial bideposited film Figure 1a shows a cross-section scanning electron micrograph (SEM) of a 174±5-nm thin film comprising upright nanorods fabricated with the SBD method. Both collimated vapours of Ta 2 O 5 were directed at an angle θ ν =75° with respect to the normal ( z axis) to the substrate plane ( xy plane). The cross-sectional dimensions of the nanorods being much smaller than the wavelength, the thin film is an optical continuum that presents an equivalent refractive index n x to normally incident light whose electric field vector vibrates along the x axis, but the equivalent refractive index changes to n y when that electric field vector vibrates along the y axis. Figure 1b shows the wavelength dependences of n x and n y , obtained by fitting these two parameters to measured data on optical transmittance [25] , [26] . The nanorod array is thus effectively birefringent, and the weak dependence of the refractive index difference n y − n x of the chosen material (Ta 2 O 5 ) on the wavelength over the 400–700 nm range simplifies the design of achromatic waveplates. Figure 1: The structure and equivalent refractive indexes of a serial bideposited Ta 2 O 5 nanorod array. ( a ) Cross-sectional scanning electron micrograph of an array of upright Ta 2 O 5 nanorods produced using the SBD method. Each collimated vapour produced a 5-nm growth, the total thickness of the nanorod array being 174±5 nm. Scale bar, 100 nm. ( b ) Equivalent refractive indexes n x (red line) and n y (blue line) of this array in the visible regime. 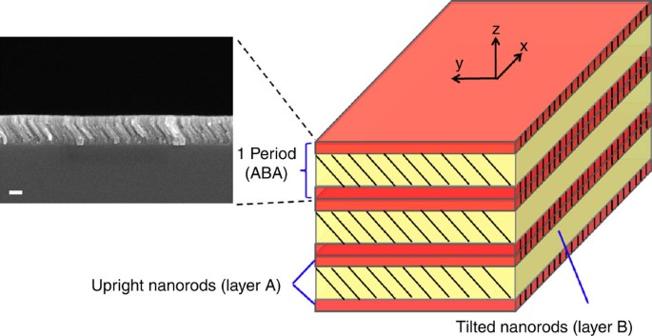Figure 2: Schematic of a unit cell ABA. Cross-sectional SEM of a unit cell ABA with a thickness of 246±5 nm. Scale bar, 100 nm. Layer A comprising upright nanorods and layer B comprising tilted nanorods form the unit cell of a periodic multilayered structure. Full size image Periodic multilayered structures For that purpose, the achromatic waveplate was conceived as a PMS, as shown in Figure 2 . The unit cell comprising three layers, with two layers labelled A sandwiching a layer labelled B, is symmetric. Layers labelled A are to be fabricated using the SBD method, with both collimated vapours oriented in the xz plane. Layers labelled B are to be fabricated using the OAD method with just a single collimated vapour oriented in the yz plane. The anisotropic optical properties of layers A and B are represented as polarization-dependent refractive indexes ( i =A, B; j =x, y). Figure 2: Schematic of a unit cell ABA. Cross-sectional SEM of a unit cell ABA with a thickness of 246±5 nm. Scale bar, 100 nm. Layer A comprising upright nanorods and layer B comprising tilted nanorods form the unit cell of a periodic multilayered structure. Full size image For normally incident light, a symmetric unit cell is equivalent to a homogeneous layer of refractive index and phase thickness (which is 2 π times the product of the refractive index and the thickness divided by the wavelength for a homogeneous thin film) [5] ; the superscript E stands for equivalent. A PMS comprising m identical symmetric unit cells is equivalent to a homogeneous layer with a refractive index and phase thickness The PMS reflects strongly in a wavelength regime called the stop band, wherein has an imaginary part. Outside the stop band, is real and the PMS can be transparent in a wavelength regime called a pass band. The parameters and are two different functions of wavelength and four other parameters ( , d A and d B ). The relationship between and departs from the simple linear relationship for a homogeneous thin film. For an achromatic waveplate, the parameters and d A,B have thus to be realized in such a way that the phase retardation m is independent of the wavelength; specifically, the differences do not have to be linearly proportional to the wavelength. The aciculate morphology of the waveplate is optically similar to the microvillar array in R8 cells of stomatopod crustaceans, and the form birefringences of the two different types of layers in the unit cell ABA of the PMS can be combined to achieve achromatic phase retardation. Three-cell PMS achromatic waveplate For this study, layers A and B were first independently deposited. The thicknesses of layers A and B were controlled to be 48±2 and 150±2 nm, respectively, and the average cross-sectional diameters of the nanorods were 26±2 nm. By varying θ ν from 65° to 80°, were experimentally found to vary from (1.663, 1.788) to (1.396, 1.451) at 632.8 nm wavelength. Likewise, at the same wavelength varied from (1.816, 1.792) to (1.458, 1.431) when θ ν was varied from 60° to 80°. The parameterized dependences of on θ ν at 632.8 nm wavelength were determined as follows: These relationships were used for designing PMS. For fabricating a PMS, θ ν was chosen as 75° for layer A so that =(1.453, 1.547) at 632.8 nm wavelength; likewise, θ ν was chosen as 70° for layer B so that =(1.662, 1.636) at the same wavelength. 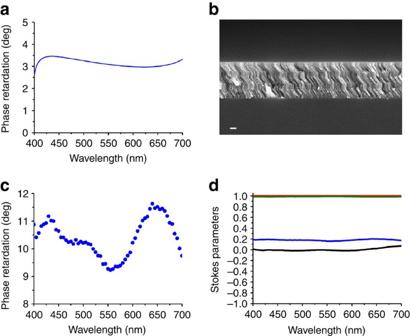Figure 3: Achromatic waveplate with a three-cell PMS. (a) Calculated spectrum of the phase retardationof the unit cell ABA on glass. (b) Cross-sectional SEM of a PMS of three unit cells, the calculated optical properties of each unit cell being presented in (a). Scale bar, 100 nm. (c) Measured spectrum of the phase retardation of the three-cell PMS on glass. (d) Measured spectra of the four Stokes parameters S0(red line), S1(black line), S2(green line) and S3(blue line) of the light transmitted by the three-cell PMS of (b), when the incident light is linearly polarized at 45° to thexaxis in thexyplane. The calculated phase retardation of the unit cell ABA on glass is 3.35±0.52° in the visible regime, as shown in Figure 3a . Figure 3: Achromatic waveplate with a three-cell PMS. ( a ) Calculated spectrum of the phase retardation of the unit cell ABA on glass. ( b ) Cross-sectional SEM of a PMS of three unit cells, the calculated optical properties of each unit cell being presented in ( a ). Scale bar, 100 nm. ( c ) Measured spectrum of the phase retardation of the three-cell PMS on glass. ( d ) Measured spectra of the four Stokes parameters S 0 (red line), S 1 (black line), S 2 (green line) and S 3 (blue line) of the light transmitted by the three-cell PMS of ( b ), when the incident light is linearly polarized at 45° to the x axis in the xy plane. Full size image Next, a PMS made of m =3 unit cells ABA was fabricated on a glass (BK7) substrate, and the phase retardation was measured over the visible regime. Figure 3b shows a cross-sectional SEM of the fabricated PMS, and Figure 3c shows that the phase retardation is 10.41±1.16° over the 400–700 nm wavelength regime. The phase retardation is thrice the value predicted in Figure 3a for a single unit cell, and the achromaticity of the three-cell PMS compares favourably with that reported for the R8 cells of stomatopod crustaceans (for which the phase retardation has a ±2.7° variation [10] ). Furthermore, the maximum variation in the phase retardation does not increase as fast as m . The polarization state of light is comprehensively captured by four quantities called the Stokes parameters [27] . For normally incident light that is linearly polarized at 45° to the x axis in the xy plane, the Stokes parameters of the light transmitted by the three-cell PMS were measured over the visible regime. As shown in Figure 3d , all four Stokes parameters are remarkably uniform over the 400–700 nm wavelength range, thereby confirming the achromaticity of the three-cell PMS. 23-cell PMS achromatic waveplate. Although the phase retardation of the three-cell PMS is 10.41°, higher values of the phase retardation can be realized by cascading several different PMS′s. Alternatively, a single m -cell PMS with high m can be designed. 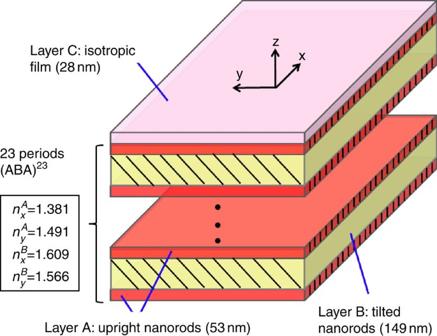Figure 4 Schematic of a 23-cell PMS with an index-matching layer at the entry pupil. Figure 4 shows the design of a 23-cell PMS that is predicted to deliver a phase retardation of 89.33° in the visible regime. Each ABA unit cell comprises layers of type A ( d A =53 nm, θ ν =78°) and B ( d B =149 nm, θ ν =73°). Layer C, made of SiO 2 , was added at the entry pupil. Figure 4 Schematic of a 23-cell PMS with an index-matching layer at the entry pupil. Full size image Calculated spectra of and of the unit cell ABA are shown in Fig. 5a . The phase retardation of a single unit cell on glass is 3.97±0.57° over the visible regime. 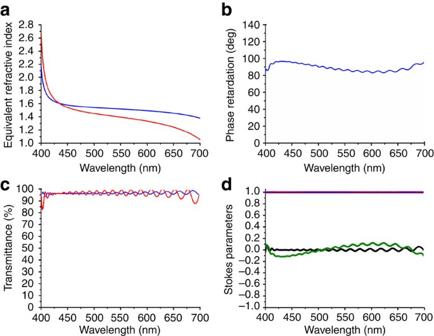Figure 5: Achromatic waveplate with a 23-cell PMS. (a) Computed spectra ofandof the unit cell ABA presented inFigure 4. (b) Computed spectrum of the phase retardation of a 23-cell PMS on glass. (c) Computed transmittance spectra of the device presented inFigure 4. (d) Computed spectra of the four Stokes parameters S0(red line), S1(black line), S2(green line) and S3(blue line) of the transmitted light of the device presented inFigure 4, when the incident light is linearly polarized at 45° to thexaxis in thexyplane. The calculated spectrum of the phase retardation of the 23-cell PMS on glass is shown in Figure 5b . The phase retardation is 89.33±6.83° over the visible regime, with a maximum variation less than thrice that of the R8 cell of a stomatopod crustacean [10] . Figure 5: Achromatic waveplate with a 23-cell PMS. ( a ) Computed spectra of and of the unit cell ABA presented in Figure 4 . ( b ) Computed spectrum of the phase retardation of a 23-cell PMS on glass. ( c ) Computed transmittance spectra of the device presented in Figure 4 . ( d ) Computed spectra of the four Stokes parameters S 0 (red line), S 1 (black line), S 2 (green line) and S 3 (blue line) of the transmitted light of the device presented in Figure 4 , when the incident light is linearly polarized at 45° to the x axis in the xy plane. Full size image Finally, an isotropic index-matching layer of SiO 2 (layer C: d C =28 nm, at 632.8 nm wavelength) was added at the entry pupil, as shown in Figure 4 . The calculated transmittance spectra for both linear polarization states, shown in Figure 5c , are very close to each other. Computed spectra of the four Stokes parameters presented in Figure 5d confirm achromaticity over the visible regime. By providing index-matching layers [28] at the entry pupil of an m -cell PMS, the overall transmittance can be made very high and quite independent of the polarization state of incident light, as shown in Figure 5 . Thus, the achromatic arrangement can be used as a drop-in device to change the polarization state of light. Our study has established achromatic phase retardation over the visible regime—an extremely rare optical property hitherto reported only in the eyes of a certain stomatopod crustacean and never before realized artificially—in a PMS with a symmetric unit cell fashioned from layers of upright and tilted Ta 2 O 5 nanorods. The artificial bioinspired device can be used to change the polarization of light over the entire visible range. Achromatic waveplates can be similarly realized for operation in different wavelength regimes. The fabrication technique for the PMS is a workhorse technique in the thin-film industry [5] , [6] , does not require expensive lithography equipment [12] , [13] , and is compatible with planar technology commonplace in electronics and optoelectronics industries. Further optimization will reduce the maximum variation in phase retardation over the visible regime, without compromising the insensitivity of the transmittance to the polarization state and the wavelength of incident light. Electron beam evaporation For the SBD method, two collimated vapours of Ta 2 O 5 were produced by electron-beam impingement of two Ta 2 O 5 targets in a vacuum chamber, wherein the base pressure was 4×10 −6 Torr. The vapours were directed onto a glass substrate (BK7) at an average angle θ ν with respect to the normal ( z axis) to the substrate plane ( xy plane), the sources of the collimated vapours being located on opposite ends of the x axis in the xz plane. Each source was located at 30 cm from the centre of the substrate plane. The cross-sectional dimensions of the substrate were 21 mm×23 mm. The OAD and SBD methods usually produce thin films with uniformity at these length scales [29] . The deposition rate was typically 0.3 nm s −1 . For the OAD method, only one of the two targets was used. Optical measurements With linearly polarized incident light, the transmittance was measured using the VASE ellipsometer (J.A. Woollam Co.). Both the phase retardation and the Stokes parameters of the transmitted light were also measured with the same equipment. All optical measurements were performed at the centre of the sample, as well as at two points diametrically apart from the centre at a distance of 10 mm from each other. The spectra of phase retardation and the Stokes parameters of the transmitted light at either of those two points on a three-cell PMS shifted by about 10 nm with respect to their counterparts obtained at the centre of the sample, thereby indicating acceptable uniformity over a circular area of 10 mm diameter. The substrate dimensions can be scaled up if the distance between the vapour source and the centre of the substrate is also increased proportionally [16] , and uniformity over larger length scales can be realized in scaled-up systems. With the angle of incidence varying over a ±5° range from normal incidence, the phase retardation was found to vary <1%. Measurements were made repeatedly at 22 °C and 24% relative humidity. The phase retardation remained the same from 2 to 72 h after fabrication. Using a sensitive polarization conversion method [30] , we found that all three principal refractive indexes of a Ta 2 O 5 thin film did not vary from 1 to 144 h after fabrication. How to cite this article: Jen Y.-J. et al . Biologically inspired achromatic waveplates for visible light. Nat. Commun. 2:363 doi: 10.1038/ncomms1358 (2011).